Tracing back the nascence of a new sex-determination pathway to the ancestor of bees and ants In several Hymenoptera, sexual fate is determined by the allelic composition at the complementary sex-determiner locus, a sex-determination mechanism that can strongly affect population dynamics. To date, the molecular identification of complementary sex determiner has only been achieved in the honeybee, where the complementary sex-determiner gene was reported to have arisen from duplication of the feminizer gene. Strikingly, the complementary sex-determiner gene was also proposed to be unique to the honeybee lineage. Here we identify feminizer and complementary sex-determiner orthologues in bumble bees and ants. We further demonstrate that the duplication of feminizer that produced complementary sex determiner occurred before the divergence of Aculeata species (~120 Myr ago). Finally, we provide evidence that the two genes evolved concertedly through gene conversion, complementary sex-determiner evolution being additionally shaped by mosaic patterns of selection. Thus, the complementary sex-determiner gene likely represents the molecular basis for single locus-complementary sex determination in the Aculeata infra-order, and possibly, in the entire Hymenoptera order. Sex determination in insects is controlled by a cascade of regulatory genes that always ends with splicing regulation of the doublesex (dsx) transcription factor by the transformer (tra)/feminizer (fem) factor [1] . In contrast, the upstream key primary signal differs among species. In several Hymenoptera (ants, bees and wasps), which are haplodiploid as 20% of the animal kingdom, it relies on the single-locus complementary sex-determination (sl-CSD) mechanism [2] : males are usually haploid, and therefore, hemizygous at the complementary sex-determiner ( csd ) locus, whereas females are diploid and heterozygous. Strikingly, diploid individuals homozygous for csd develop into males that are usually sterile, possibly driving bottlenecked populations towards extinction [3] , [4] . The csd gene was first cloned in the honeybee, Apis mellifera , where it was elegantly shown to be the primary allelic signal [5] , [6] , ensuring female-specific splicing of fem in response to heterozygosity at csd [1] . Furthermore, csd was suggested to result from a recent duplication of fem that occurred after the divergence of stingless bees, bumble bees and honeybees (~70 Myr ago) and before that of honeybees (~10 Myr ago) [6] . This assumption was based on analyses showing that fem sequences of four honeybee species cluster together, separately from csd sequences, and on the failure to identify any csd orthologue in the Bombus terrestris bumble bee genome, using a bioinformatic approach [6] . Hence, csd was considered as unique to the honeybee lineage and unlikely to represent the 'universal' molecular basis of sl-CSD in Hymenoptera. In this work, we provide evidence from bioinformatic analyses and gene-expression data that published bumble bee and ant genomes contain fem and csd orthologues, and we unravel the mechanisms underlying their evolution. On the basis of our findings, csd likely represents the molecular basis for sl-CSD in Aculeata species, and possibly in all Hymenoptera. Identification and organization of hymenopteran fem and csd genes Identification of potentially functional orthologues of csd and fem was performed in available bumble bee genomes ( Bombus terrestris , Bombus impatiens ), as well as in almost all recently released ant genomes ( Atta cephalotes , Camponotus floridanus , Harpegnathos saltator , Solenopsis invicta , Acromyrmex echinatior, Linepithema humile , Pogonomyrmex barbatus) . Full-length coding sequences with high similarity to the female-specific A. mellifera fem coding sequence were inferred through BLAST analyses and manual adjustment of the exon boundaries ( Fig. 1a ; Supplementary Tables S1 and S2 ). All fem and csd paralogues share more than 80% identity in their coding sequences and have a conserved protein domain organization ( Fig. 1b ; Supplementary Fig. S1 and Table S3 ). Because of the incompleteness of some genome assemblies, a few sequence identifications remained partial or ambiguous. In L. humile , only the first four coding exons of fem and csd were localized. Although we could not identify csd in S. invicta , a duplication of fem , named TraB , was previously reported in this species in the opposite direction to fem [7] . Finally, the apparent lack of csd in A. echinatior ( [8] and our analysis) requires further clarification. 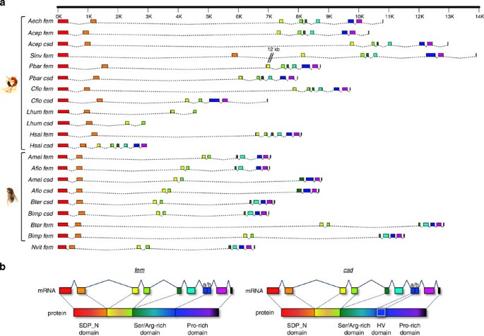Figure 1:femandcsdexon–intron organization. (a)fem- andcsd-coding exons (boxes) are represented at scale, except forS. invicta femin which 12 kb are condensed. Homologous coding exons are indicated by the same colour. ForL. humile femandcsd, only the first four coding exons were identified. Genes are listed according to the phylogenies (Fig. 5a;Supplementary Fig. S2). (b) The domain organization of Fem and Csd proteins and the corresponding exons in the coding sequences are represented. Both proteins contain the SDP_N (sex-determiner protein amino-terminal) domain encoded by exons 1+2, the serine/arginine (Ser/Arg)-rich domain encoded by exons 5+6+7a, and the proline (Pro)-rich domain encoded by exons 7b+8+9. Csd proteins also contain a hypervariable (HV)-domain encoded by exon 7a. Abbreviations:Amel,Apis mellifera;Aflo,Apis florea;Bter,Bombus terrestris;Bimp,Bombus impatiens;Aech,Acromyrmex echinatior;Acep,Atta cephalotes;Pbar,Pogonomyrmex barbatus;Hsal,Harpegnathos saltator;Cflo,Camponotus floridanus;Sinv,Solenopsis invicta;Lhum,Linepithema humile;Nvit,Nasonia vitripennis; mRNA, messenger RNA. Figure 1: fem and csd exon–intron organization. ( a ) fem - and csd -coding exons (boxes) are represented at scale, except for S. invicta fem in which 12 kb are condensed. Homologous coding exons are indicated by the same colour. For L. humile fem and csd , only the first four coding exons were identified. Genes are listed according to the phylogenies ( Fig. 5a ; Supplementary Fig. S2 ). ( b ) The domain organization of Fem and Csd proteins and the corresponding exons in the coding sequences are represented. Both proteins contain the SDP_N (sex-determiner protein amino-terminal) domain encoded by exons 1+2, the serine/arginine (Ser/Arg)-rich domain encoded by exons 5+6+7a, and the proline (Pro)-rich domain encoded by exons 7b+8+9. Csd proteins also contain a hypervariable (HV)-domain encoded by exon 7a. Abbreviations: Amel , Apis mellifera ; Aflo , Apis florea ; Bter , Bombus terrestris ; Bimp , Bombus impatiens ; Aech , Acromyrmex echinatior ; Acep , Atta cephalotes ; Pbar , Pogonomyrmex barbatus ; Hsal , Harpegnathos saltator ; Cflo , Camponotus floridanus ; Sinv , Solenopsis invicta ; Lhum , Linepithema humile ; Nvit , Nasonia vitripennis ; mRNA, messenger RNA. Full size image In silico prediction of the occurrence of fem and csd sequences in bumble bees and ants was further confirmed by demonstrating their expression in vivo . Indeed, RT–PCR, using specific primers, allowed amplifying complementary DNA fragments corresponding to fem and csd in individuals from one bumble bee species, B. terrestris , and two ant species, H. saltator and C. floridanus ( Fig. 2 ). fem PCR products from females were of the predicted size in the three species, while larger products were obtained from males in B. terrestris and H. saltator , corresponding to male-specific splice variants, coding for truncated Fem proteins. In C. floridanus , no fem cDNA could be amplified in males in our RT–PCR conditions. Regarding csd , PCR fragments were of the expected size and identical in males and females of the three species. fem and csd expression is thus consistent with data from A. mellifera [5] that is, the absence of a functional Fem protein in males and the production of an identical Csd protein in both sexes. Therefore, it can reasonably be assumed that these genes ensure functions similar to those reported in the honeybee. Overall, the unambiguous identification of at least six csd orthologues outside the honeybee lineage, the expression of which was confirmed in bumble bee and ant species, demonstrates that csd is not unique to the honeybee lineage. 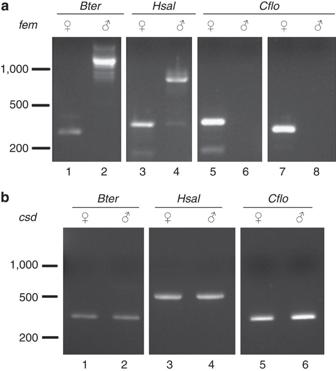Figure 2:femandcsdexpression in bumble bee and ants. (a) Identification offemtranscripts by RT–PCR inB. terrestris(Bter),H. saltator(Hsal), andC. floridanus(Cflo) female (♀) and male (♂) individuals. PCR was carried out using species-specificfemprimers chosen on distinct exons. PCR products of expected size and sequence, coding for the predicted female Fem proteins were obtained in females. In males, larger PCR products were obtained inB. terrestrisandH. saltator, corresponding to alternative splice variants that include male specific exons and encode truncated Fem proteins. In theC. floridanusmale, no PCR product was obtained with two primer pairs (lanes 6 and 8). (b) Identification ofcsdtranscripts by RT–PCR in the same individuals as in A, using species-specificcsdprimers on distinct exons. Size markers (in base pairs) are indicated. Primer pairs used in the indicated lanes are provided inSupplementary Table S7. Figure 2: fem and csd expression in bumble bee and ants. ( a ) Identification of fem transcripts by RT–PCR in B. terrestris ( Bter ), H. saltator ( Hsal ), and C. floridanus ( Cflo ) female (♀) and male (♂) individuals. PCR was carried out using species-specific fem primers chosen on distinct exons. PCR products of expected size and sequence, coding for the predicted female Fem proteins were obtained in females. In males, larger PCR products were obtained in B. terrestris and H. saltator , corresponding to alternative splice variants that include male specific exons and encode truncated Fem proteins. In the C. floridanus male, no PCR product was obtained with two primer pairs (lanes 6 and 8). ( b ) Identification of csd transcripts by RT–PCR in the same individuals as in A, using species-specific csd primers on distinct exons. Size markers (in base pairs) are indicated. Primer pairs used in the indicated lanes are provided in Supplementary Table S7 . Full size image We could determine the relative positions of fem and csd in most species, showing that csd localizes downstream or upstream fem , in the same or opposite orientation, depending on the species ( Fig. 3 ). The distance between fem and csd ranges from 1.8 kb ( P. barbatus) to >176.2 kb ( B. impatiens ). In Bombus species, csd localizes in unplaced scaffolds, 6.5 kb upstream the LIN1-like gene, which lies about 2.2 Mb upstream fem in A. mellifera ( Fig. 4 ). The size of fem and csd genes also varies between species owing to huge differences in intron lengths ( Fig. 1a ), including intragenic duplications, some of which being likely at the origin of the male-specific exons in A. mellifera (not shown). Together, these findings evidence frequent genomic reorganizations of the sex-determining locus, as already reported in A. mellifera [9] . 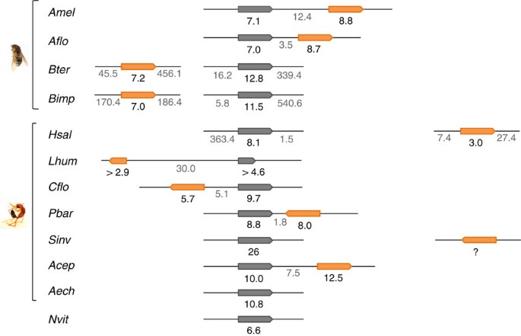Figure 3: Diagram of relative genomic positions offemandcsd. Relative genomic positions and orientations (arrowheads in 5′-to-3′ direction) of inferredfem(grey arrows) andcsd(orange arrows) genes are represented. Afemduplicate (question mark) was reported inS.invicta7, but not found in our analysis. Gene sizes (in kb, bold numbers) do not include the 5′ and 3′ untranslated regions. Intergenic distances or minimum distances surrounding the genes (when the genes were found in distinct scaffolds) are indicated (in kb). Abbreviations:Amel,Apis mellifera;Aflo,Apis florea;Bter,Bombus terrestris;Bimp,Bombus impatiens;Aech,Acromyrmex echinatior;Acep,Atta cephalotes;Pbar,Pogonomyrmex barbatus;Hsal,Harpegnathos saltator;Cflo,Camponotus floridanus;Sinv,Solenopsis invicta;Lhum,Linepithema humile;Nvit,Nasonia vitripennis. Figure 3: Diagram of relative genomic positions of fem and csd . Relative genomic positions and orientations (arrowheads in 5′-to-3′ direction) of inferred fem (grey arrows) and csd (orange arrows) genes are represented. A fem duplicate (question mark) was reported in S.invicta [7] , but not found in our analysis. Gene sizes (in kb, bold numbers) do not include the 5′ and 3′ untranslated regions. Intergenic distances or minimum distances surrounding the genes (when the genes were found in distinct scaffolds) are indicated (in kb). Abbreviations: Amel , Apis mellifera ; Aflo , Apis florea ; Bter , Bombus terrestris ; Bimp , Bombus impatiens ; Aech , Acromyrmex echinatior ; Acep , Atta cephalotes ; Pbar , Pogonomyrmex barbatus ; Hsal , Harpegnathos saltator ; Cflo , Camponotus floridanus ; Sinv , Solenopsis invicta ; Lhum , Linepithema humile ; Nvit , Nasonia vitripennis . 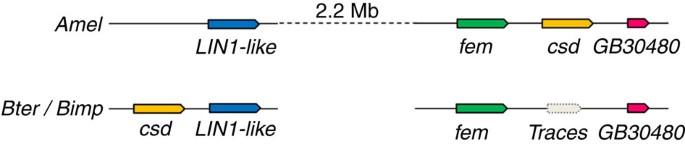Figure 4: Comparison of genomic regions containingfemandcsdinBombusandApisspecies. Schematic representation of the relative positions and orientations offem,csd, and nearby genes calledGB30480andLIN1-like(boxes with arrowhead in 5′ to 3′ direction). InA. mellifera(Amel),csdlocalizes downstreamfemand upstreamGB30480. InB. terrestris(Bter) andB. impatiens(Bimp), the analogous region (traces) contains sequence similarities with up to 82% identity with parts of thefemsequence, between exons 3 and 9, but regions homologous to exons 1+2 are absent. InBombus,csdlocalizes in a distinct scaffold, upstreamLIN1-like, which is found 2.2 Mb upstreamfeminA. mellifera. Full size image Figure 4: Comparison of genomic regions containing fem and csd in Bombus and Apis species. Schematic representation of the relative positions and orientations of fem , csd , and nearby genes called GB30480 and LIN1-like (boxes with arrowhead in 5′ to 3′ direction). In A. mellifera ( Amel ), csd localizes downstream fem and upstream GB30480 . In B. terrestris ( Bter ) and B. impatiens ( Bimp ), the analogous region (traces) contains sequence similarities with up to 82% identity with parts of the fem sequence, between exons 3 and 9, but regions homologous to exons 1+2 are absent. In Bombus , csd localizes in a distinct scaffold, upstream LIN1-like , which is found 2.2 Mb upstream fem in A. mellifera . Full size image Phylogeny of fem and csd genes We then carried out phylogenetic analyses, using fem and csd nucleotide and protein sequences, to determine evolutionary relationships. Nasonia vitripennis , whose genome is sequenced and contains fem but not csd sequences [10] , was used as an outgroup. This species does not use a CSD-based sex-determination mechanism, but relies on maternal imprinting of the tra/fem gene to ensure male or female development. Tree topologies ( Fig. 5 ; Supplementary Fig. S2 ) were congruent with the current classification of Hymenoptera, except for N. vitripennis fem that clusters with fem of bees, suggesting a higher evolutionary rate of fem in ants compared with bees. fem and csd sequences cluster separately inside the bumble bee and honeybee genera, as previously reported for the honeybee [6] , suggesting independent duplications of fem at the origin of csd in the two lineages. In ants, where only one genome is available per genus, fem and csd paralogues cluster together, also suggesting independent duplications ancestral to each genus. However, this hypothesis of recurrent duplications at the fem locus is clearly not parsimonious when considering the high number of independent duplications that would have occurred (at least six in our analysis). Besides, no more than two paralogues were found in each genome, and no traces of degenerate copies of ancestral fem duplications were identified, except in bumble bees. Therefore, we considered the alternative hypothesis of one ancestral duplication event, followed by concerted evolution of the fem/csd loci. 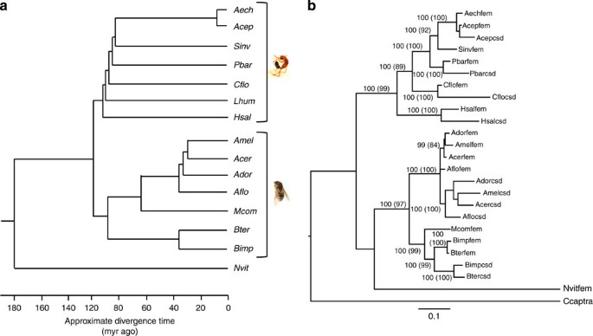Figure 5: Phylogenetic analysis offemandcsdcoding sequences. (a) Phylogeny31,32,33of the Hymenopteran species investigated in this study. (b) Bayesian phylogenetic tree offemandcsdcoding sequences of hymenopteran species and of the DipteranCeratitis capitata fem-homologuetransformer(Ccaptra). The same tree topology was obtained using maximum likelihood inference; node supports are shown by posterior probabilities >90% for the Bayesian method and bootstrap values >80% for the maximum likelihood method (brackets). The scale bar represents the estimated number of substitutions per site. Abbreviations:Amel,Apis mellifera;Aflo,Apis florea;Acer, Apis cerana;Ador, Apis dorsata; Bter,Bombus terrestris;Bimp,Bombus impatiens; Mcom, Melipona compressipes; Aech,Acromyrmex echinatior;Acep,Atta cephalotes;Pbar,Pogonomyrmex barbatus;Hsal,Harpegnathos saltator;Cflo,Camponotus floridanus;Sinv,Solenopsis invicta;Lhum,Linepithema humile;Nvit,Nasonia vitripennis. Figure 5: Phylogenetic analysis of fem and csd coding sequences. ( a ) Phylogeny [31] , [32] , [33] of the Hymenopteran species investigated in this study. ( b ) Bayesian phylogenetic tree of fem and csd coding sequences of hymenopteran species and of the Dipteran Ceratitis capitata fem -homologue transformer ( Ccaptra ). The same tree topology was obtained using maximum likelihood inference; node supports are shown by posterior probabilities >90% for the Bayesian method and bootstrap values >80% for the maximum likelihood method (brackets). The scale bar represents the estimated number of substitutions per site. Abbreviations: Amel , Apis mellifera ; Aflo , Apis florea ; Acer, Apis cerana ; Ador, Apis dorsata; Bter , Bombus terrestris ; Bimp , Bombus impatiens; Mcom, Melipona compressipes; Aech , Acromyrmex echinatior ; Acep , Atta cephalotes ; Pbar , Pogonomyrmex barbatus ; Hsal , Harpegnathos saltator ; Cflo , Camponotus floridanus ; Sinv , Solenopsis invicta ; Lhum , Linepithema humile ; Nvit , Nasonia vitripennis . Full size image The presence of a degenerate, non-functional copy of fem about 20 kb downstream fem in both bumble bee species ( Fig. 4 ) was intriguing. However, it may be easily explained under the fem single ancestral duplication hypothesis, given the major chromosomal reorganizations that occurred in B. terrestris since its divergence from A. mellifera [11] . Indeed, in the Bombus lineage, the non-functional copy may correspond to the ancestral duplication of fem whereas the distantly located csd would result from a secondary reorganization event that led to creation of a functional distant copy (that is, csd ) while the ancestral copy degenerated. However, a second independent duplication of fem specific to the bumble bee lineage cannot be excluded. Concerted evolution between fem and csd Concerted evolution is a universal phenomenon of intraspecies sequence homogenization leading to higher sequence similarity of paralogues compared with orthologues [12] , [13] , [14] , [15] . The two molecular mechanisms underlying concerted evolution are unequal crossing-over and gene conversion. Whereas unequal crossing-over usually applies to multigene families, with copy-number variations and tandem 'head-to-tail' arrangement, gene conversion is the non-reciprocal transfer of DNA fragments, generally <1 kb in size, usually occurring in specific regions of duplicated genes that are functionally related. The use of the GENECONV program (that detects both mechanisms) allowed us to identify a total of 28 conversion tracts between the fem / csd paralogues in eight species ( Fig. 6a ; Supplementary Table S4 ). The conversion tracts are mostly <1 kb and 50% of them involve two or more neighbouring exons and the intron(s) in between. Intron-covering conversion tracts correspond to exons 1+2 (encoding the conserved SDP_N domain), exons 3+4, and exons 7b+8+9 (encoding the conserved proline-rich domain) ( Fig. 1b ; Supplementary Fig. S1 ). Significantly, conversion tracts never include exon 5, and they include exons 6+7a only in three species, suggesting a low rate of sequence homogenization in the corresponding arginine/serine-rich variable domain that accounts for csd allelic diversity. The sequence similarity between fem and csd paralogues would thus result from concerted evolution through gene conversion, likely ensuring conservation of functionally important domains. Importantly, the observation that the fem/csd phylogeny is congruent with the real history of the genes, at the species level, within the Apis and Bombus lineages, but not at the level of Bombus , Apis and ant genera ( Fig. 5 ; Supplementary Fig. S2 ) perfectly fits Innan's predictions for genes undergoing concerted evolution [15] , that is, that the probability to observe phylogenetic incongruence is negatively correlated with the time between the duplication and the speciation events. In agreement with this model, fem and csd cluster separately within the Apis and Bombus lineages (leading to a congruent phylogeny) owing to a longer time between the ancestral fem duplication and the speciation events in these lineages, compared with that between the fem duplication and the separation of the different genera. 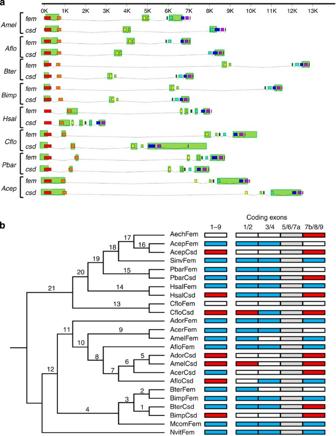Figure 6: Evolution offemandcsdgenes. (a) Intraspecies gene conversion tracts betweenfemandcsd(green boxes). The analysis was performed on sequence alignments corresponding to subdivisions of the coding sequence (exons 1+2, exons 3+4, exons 3–9, exons 5–9) including intron sequences (up to 500 nucleotides) up- and downstream the outermost exons. When totally overlapping conversion tracts were identified, only the longest was retained. Partially overlapping conversion tracts were all retained. (b) Positive selection analysis. The cladogram is based on the Fem and Csd protein phylogeny (Fig. 5). Branches are numbered (1 to 21) and Ka/Ks values for each branch are given inSupplementary Table S6. Occurrence of positive selection (ratios of non-synonymous versus synonymous (Ka/Ks) amino acid substitutions >1, with a posterior probability of Ka>Ks greater than 95%) is indicated for the entire coding sequences (exons 1-9) and four subdivisions thereof (red boxes). Exon 7 is divided into 7a (5′ hypervariable part) and 7b (3′ conserved part). Regions with Ka/Ks values <1 and a probability of Ka>Ks lower than 1% are also represented (blue boxes). Abbreviations:Amel,Apis mellifera;Aflo,Apis florea;Acer, Apis cerana;Ador, Apis dorsata; Bter,Bombus terrestris;Bimp,Bombus impatiens; Mcom, Melipona compressipes; Aech, Acromyrmex echinatior; Acep, Atta cephalotes; Pbar, Pogonomyrmex barbatus;Hsal,Harpegnathos saltator;Cflo,Camponotus floridanus;Sinv,Solenopsis invicta;Nvit,Nasonia vitripennis. Figure 6: Evolution of fem and csd genes. ( a ) Intraspecies gene conversion tracts between fem and csd (green boxes). The analysis was performed on sequence alignments corresponding to subdivisions of the coding sequence (exons 1+2, exons 3+4, exons 3–9, exons 5–9) including intron sequences (up to 500 nucleotides) up- and downstream the outermost exons. When totally overlapping conversion tracts were identified, only the longest was retained. Partially overlapping conversion tracts were all retained. ( b ) Positive selection analysis. The cladogram is based on the Fem and Csd protein phylogeny ( Fig. 5 ). Branches are numbered (1 to 21) and Ka/Ks values for each branch are given in Supplementary Table S6 . Occurrence of positive selection (ratios of non-synonymous versus synonymous (Ka/Ks) amino acid substitutions >1, with a posterior probability of Ka>Ks greater than 95%) is indicated for the entire coding sequences (exons 1-9) and four subdivisions thereof (red boxes). Exon 7 is divided into 7a (5′ hypervariable part) and 7b (3′ conserved part). Regions with Ka/Ks values <1 and a probability of Ka>Ks lower than 1% are also represented (blue boxes). Abbreviations: Amel , Apis mellifera ; Aflo , Apis florea ; Acer, Apis cerana ; Ador, Apis dorsata; Bter , Bombus terrestris ; Bimp , Bombus impatiens; Mcom, Melipona compressipes; Aech, Acromyrmex echinatior; Acep, Atta cephalotes; Pbar, Pogonomyrmex barbatus ; Hsal , Harpegnathos saltator ; Cflo , Camponotus floridanus ; Sinv , Solenopsis invicta ; Nvit , Nasonia vitripennis . Full size image An alternative explanation for sequence homogenization between paralogues would be strong purifying selection [13] , [16] , [17] . Even though this hypothesis is unlikely given the high proportion of intron-covering conversion tracts, we investigated the proportion of synonymous nucleotide differences (Ps) for all paralogues and orthologues ( Supplementary Table S5 ). Under strong purifying selection without gene conversion, high Ps values are expected. In ants, Ps values are lower for paralogues compared with orthologues indicating strong concerted evolution. In the Apis and Bombus genera, Ps values are lower for paralogues compared with orthologues from distinct genera, but not compared with orthologues within the same genus; that is, concerted evolution is detected between, but not within, genera. In addition to clarifying phylogenetic data, this suggests that the conversion events preceded the divergence within the honeybee and bumble bee lineages, in agreement with conversion tract similarities within these genera ( Fig. 6a ). csd genes evolve under a mosaic pattern of selective forces Further analysis of non-synonymous substitutions per site (Ka) versus synonymous substitutions per site (Ks) demonstrates that all investigated csd genes evolve under positive selection (Ka/Ks>1) ( Fig. 6b ; Supplementary Table S6 ) as already reported for the honeybee lineage [6] . Because gene-sequence parts may evolve under different selection pressures, we investigated Ka/Ks values in subdivisions of the coding sequences that best fitted domain localizations and gene-conversion tracts. Exons 5+6+7a, encoding most of the arginine/serine-rich variable domain, were omitted from this analysis because of their low level of sequence conservation and the high proportion of gaps in the alignment ( Supplementary Fig. S3 ). Interestingly, we found that csd evolves under a mosaic pattern of positive and purifying selection. Positive selection mainly shapes the proline-rich domain (exons 7b+8+9), whereas strong purifying selection operates on exons 3+4, likely ensuring conservation of the putative auto-regulatory domain. The SDP_N domain (exons 1+2) is generally under purifying selection, except for A. mellifera and C. floridanus , in which positive selection was detected. As expected, the progenitor gene fem evolves under purifying selection in all regions, consistent with its ancestral fundamental role in sex determination [1] , [6] . The fem/csd family is one of the rare convincing examples of duplication followed by neofunctionalization as a source of evolutionary novelty, here the upward growth of the sex-determining pathway [6] . Our results suggest that the complementary allele-based function of csd was likely achieved through the action of strong positive selection and the inactivation of gene conversion in parts of the gene. Most importantly, fem / csd represents a novel example of gene families evolving under this specific mosaic evolutionary pattern [17] , [18] , [19] , [20] , [21] , [22] , which may help gaining insights into the underlying functional constraints. Our work demonstrates that the csd gene is present and expressed in bumble bees and ants in addition to honeybees. Most interestingly, we provide evidence for a single ancestral duplication of fem at the origin of csd , having occurred before the divergence of Vespoidea and Apoidea (at least 120 Myr ago). We thus propose csd as a likely candidate for the molecular basis of sl-CSD in the Aculeata monophyletic group. If there is a consensus to consider that CSD is the ancestral mode of sex determination in Hymenoptera [23] , [24] , sl-CSD ancestry is still a matter of debate [2] . Indeed, several species are predicted or reported [25] to use multi-locus CSD (ml-CSD), a mechanism that involves more than one multiallelic sex-determining loci. Diploid individuals heterozygous at one or more of these loci develop into females, and the risk of developing into diploid males thus decreases with each additional sex locus. ml-CSD should therefore be less prone to the production of diploid males, which are usually of reduced fitness. The demonstration that the csd gene is the ancestral molecular basis of sl-CSD not only in honeybees, but likely in all Aculeata and possibly in all Hymenoptera, and the frequent genomic reorganizations observed at the fem/csd sex locus, make it possible to propose that ml-CSD evolved from sl-CSD through duplication of this locus. Indeed, duplications of csd would be strongly advantageous in case of reduced allelic diversity. As suggested by Asplen et al . [2] , reversion from ml-CSD to sl-CSD would be explained by fixation events at all but one locus, owing to relaxed allelic frequency-dependent selection. Final identification of the ancestral CSD mechanism in Hymenoptera will await the sequencing of more Hymenoptera genomes and the full understanding of the molecular basis of ml-CSD. Investigation of csd function and allelic diversity in Aculeata species, other than honeybees, will pave the way for major advances in the understanding of sex determination in Hymenoptera. It also constitutes a prerequisite for estimating sl-CSD impact on the decrease/extinction of bottlenecked populations. Future studies should address whether csd accounts for sl-CSD in all major subgroups of Hymenoptera ( Symphyta , Parasitica and Aculeata ) that all contain CSD-bearing species. Finally, the characterization of csd alleles might further help developing conservation strategies to maintain biodiversity, a major challenge for the many ecologically and economically important species in the Hymenoptera order. Sequence analysis BLAST with A. mellifera fem - and csd -coding sequences was carried out on Hymenoptera genome sequences available at the Hymenoptera Genome Database ( http://hymenopteragenome.org/ ) and the 'Ant Genomics Database' ( http://www.antgenomes.org/ ) websites. Sequences with high similarities were extracted and analysed with the Geneious software package ( http://www.geneious.com ) for manual adjustment of the exon boundaries. Intron/exon maps were drawn using FancyGene ( http://host13.bioinfo3.ifom-ieo-campus.it/fancygene/ ). Sequence alignments were performed using MUSCLE [26] . jModelTest [27] and ProtTest [28] were used to select the best fitting nucleotide and amino-acid substitution models, respectively. Phylogenetic trees were obtained by maximum likelihood (PhyML) and Bayesian inference (MrBayes). The detection of tree branches under positive selection was done using GA Branch in the HyPhy package [29] . Gene conversion events were identified using GENECONV [30] . Reported conversion tracts are global inner fragments with P - Sim values ≤0.05. GenBank EntrezNucleotide accession numbers are BK006346 ( Amel fem and Amel csd ), EU100937 ( Acer fem ), EU100916 ( Acer csd ), EU100939 ( Ador fem ), EU100935 ( Ador csd ), EU139305 ( Mcom fem ), XM_003402310 ( Bter fem ), NM_001134827 ( Nvit fem ), AF434936 ( CcapTra ). RT–PCR experiments Total RNA was isolated from single B. terrestris , H. saltator and C. floridanus individuals using TRIzol reagent (Ambion), treated with DNase I (Euromedex), and reverse transcribed using the Superscript II kit (Invitrogen) and oligo(dT) 15 . PCR was carried out using the GoTaq DNA polymerase (Promega) and the following PCR protocol: 2 min denaturation at 95°C, 35 cycles of denaturation at 95°C (30 s), annealing at 54–58°C (30 s) depending on the primer pairs, elongation at 72°C (90 s), and 5 min of final elongation at 72°C. fem or csd primers were designed to specifically amplify fem and csd transcripts (sequences provided in Supplementary Table S7 ), and were chosen on distinct exons to control for absence of genomic contamination. PCR products were resolved on 1.5% agarose gels in 0.5X TBE buffer and further sequenced (GATC Biotech). How to cite this article: Schmieder, S. et al . Tracing back the nascence of a new sex-determination pathway to the ancestor of bees and ants. Nat. Commun. 3:895 doi: 10.1038/ncomms1898 (2012).